NEDD4 ubiquitinates TRAF3 to promote CD40-mediated AKT activation CD40, a member of tumour necrosis factor receptor (TNFR) superfamily, has a pivotal role in B-cell-mediated immunity through various effector pathways including AKT kinase, but the signal transduction of CD40-meidated AKT activation is poorly understood. Here we report that the neural precursor cell expressed developmentally downregulated protein 4 (NEDD4), homologous to E6-AP Carboxyl Terminus family E3 ubiquitin ligase, is a novel component of the CD40 signalling complex. It has a key role in CD40-mediated AKT activation and is involved in modulating immunoglobulin class switch through regulating the expression of activation-induced cytidine deaminase. NEDD4 constitutively interacts with CD40 and mediates K63-linked ubiquitination of TNFR-associated factor3 (TRAF3). The ubiquitination of TRAF3 by NEDD4 is critical for CD40-mediated AKT activation. Thus, NEDD4 is a previously unknown component of the CD40 signalling complex necessary for AKT activation. CD40 is a member of tumour necrosis factor receptor (TNFR) superfamily that controls central events of B-cell immunity, such as immunoglobulin class switch, memory B-cell generation and germinal centre formation [1] , [2] . CD40 engagement induces assembly of a CD40 signalling complex, which mediates subsequent activation of nuclear factor κB (NF-κB) family members through the canonical and non-canonical pathways, mitogen-activated protein kinases (MAPKs) and AKT signalling pathways and results in various downstream events critical for CD40 function [3] , [4] . The formation of the primary CD40 signalling complex is achieved by recruiting multiple adaptor proteins to the receptor upon its engagment by CD40 ligand (CD40L) [5] . Among the known components of the CD40 signalling complex, several TNFR-associated factors (TRAFs) [6] , [7] , TRAF2, TRAF3 and TRAF6, bind to CD40 and mediate downstream signalling. TRAF2 and TRAF6 are involved in CD40-mediated MAPK and NF-κB activation [8] , [9] . In contrast, the role of TRAF3, the first protein identified as a component of the CD40 signalling complex, has been more obscure and controversial because CD40-mediated NF-κB and MAPK activations remain largely intact in Traf3 −/− B cells [10] . Recent reports suggest that TRAF3 negatively regulates MAPK activation and non-canonical NF-κB signalling [11] , [12] , [13] , [14] . Although CD40 is known to activate AKT signalling, and AKT has been suggested to be involved in CD40-mediated immunoglobulin class switch, the role of TRAFs in CD40-mediated AKT activation is not fully investigated [15] , [16] . Ubiquitination of TRAFs has key roles in CD40 signalling, and it has been found that both K48- and K63-linked ubiquitination of several components of the CD40 complex are involved in generation and transmission of its signals [5] , [12] . For instance, it is reported that K63-linked ubiquitination of TRAF2 in response to CD40 engagement modulates inhibitor of apoptosis protein 1/2 (cIAP1/2) activity [12] , whereas K48-linked ubiquitination of TRAF3 leads to its degradation and subsequent NF-κ-B inducing kinase (NIK) stabilization and activation [11] , [12] . But it is not clear whether TRAF3 is also subjected to K63-linked ubiquitination during CD40 signal transduction as was seen upon Toll-like receptor 3 activation [17] , [18] . Neural precursor cell-expressed developmentally downregulated gene 4 (NEDD4) is a homologous to E6-AP C-terminus (HECT) E3 ubiquitin ligase, and it is characterized by an N-terminal C2 domain, 3-4 WW repeats and a C-terminal HECT E3 ligase domain [19] . NEDD4 has been reported to have roles in various biological processes, including adaptive immunity [20] . For example, NEDD4 is involved in the regulation of growth factor receptor signalling by controlling receptor stability [21] , [22] . However, the full details of NEDD4-mediated signalling are still not clear. It was also suggested that NEDD4 regulates T-cell activation, but whether NEDD4 is involved in modulating B-cell function is unknown [20] . In our study, we identified NEDD4 as a novel component of the CD40 signalling complex. NEDD4 constitutively interacts with CD40 and mediates the K63-linked ubiquitination of TRAF3 when TRAF3 is recruited to the CD40 complex. Importantly, our data suggest that NEDD4-mediated K63-linked ubiquitination of TRAF3 is critical for CD40-mediated AKT activation, and the regulation of immunoglobulin class switch. NEDD4 is a component of the CD40 signalling complex As the regulation of CD40 signalling is not fully understood, we investigated whether there are additional previous undiscovered components of the CD40 signalling complex. To this end, the CD40 signalling complex was obtained by immunoprecipitation with a CD40 antibody from mouse B-cell lymphoma A20 cells treated or untreated with CD40L and analysed with mass spectrometry. Although no novel signal-dependent recruited protein was identified, the HECT E3 ubiquitin ligase NEDD4 was found to interact with CD40 constitutively regardless of CD40L treatment ( Supplementary Fig. 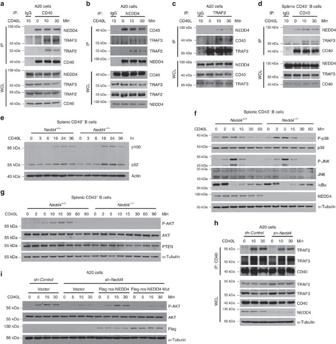Figure 1: NEDD4 is a constitutive component of the CD40 signalling complex required for AKT activation. (a–d) A20 cells were treated with CD40L (0.5 μg ml−1), and at the indicated times, cell lysates were immunoprecipitated (IP) with anti-CD40 (sc-975, Santa Cruz Biotechnology) (a,d), anti-NEDD4 (b) and anti-TRAF3 (c). The gel-separated immune complexes and whole-cell lysate (WCL) were immunoblotted with the indicated antibodies. (e–g) Primary CD43–splenic B cells were isolated from C57BL/6 mice reconstituted withNedd4+/+orNedd4−/−fetal liver stem cells and stimulated with CD40L. At the indicated times, cell lysates were collected and immunoblotted with the indicated antibodies to measure p100 processing (e), phosphorylation of MAPKs, degradation of IκBα (f), activation of AKT and PTEN expression level (g). (h) A20 cells transduced with lentiviruses containing control or NEDD4shRNAs were stimulated with CD40L. At the indicated times, cell lysates were immunoprecipitated (IP) with CD40 antibody and the co-precipited proteins were analysed by immunoblotting with the indicated antibodies. (i) Control or NEDD4shRNAs A20 cells were transfected with vector, shRNA-resistant NEDD4 (Flag-resNEDD4) or NEDD4 E3 ubiquitin ligase-dead mutant (Flag-resNEDD4Mut) as indicated. After 36 h, cell lysates were collected after CD40L stimulation for the indicated times and the expression of Flag-resNEDD4 and Flag-resNEDD4/Mut and AKT activation were examined by immunoblotting. p-, phosphorylated. Data are representative of at least three independent experiments. 1a and Supplementary Table 1 ). This finding was confirmed by Stable Isotope Labelling by Amino acids in Cell culture analysis, which revealed CD40L inducible recruitment of TRAF3 but constitutive binding of NEDD4 ( Supplementary Fig. 1b ). Furthermore, immunobloting analysis showed that CD40 and NEDD4 were co-precipitated no matter whether a CD40 or a NEDD4 antibody was used to perform the immunoprecipitation from A20 cells untreated or treated with CD40L ( Fig. 1a,b Supplementary Fig. 2 ). As controls, CD40L-induced TRAF2 and TRAF3 recruitments were detected in CD40 immunoprecipitation experiments ( Fig. 1a,b ). The presence of NEDD4 in the CD40 complex following CD40 engagement was also observed when TRAF3 was immunoprecipitated ( Fig. 1c ). More importantly, the constitutive interaction between CD40 and NEDD4 could also be detected in primary CD43 − B cells ( Fig. 1d ). These results indicated that NEDD4 binds to CD40 constitutively. Figure 1: NEDD4 is a constitutive component of the CD40 signalling complex required for AKT activation. ( a – d ) A20 cells were treated with CD40L (0.5 μg ml − 1 ), and at the indicated times, cell lysates were immunoprecipitated (IP) with anti-CD40 (sc-975, Santa Cruz Biotechnology) ( a , d ), anti-NEDD4 ( b ) and anti-TRAF3 ( c ). The gel-separated immune complexes and whole-cell lysate (WCL) were immunoblotted with the indicated antibodies. ( e – g ) Primary CD43 – splenic B cells were isolated from C57BL/6 mice reconstituted with Nedd4 +/+ or Nedd4 −/− fetal liver stem cells and stimulated with CD40L. At the indicated times, cell lysates were collected and immunoblotted with the indicated antibodies to measure p100 processing ( e ), phosphorylation of MAPKs, degradation of IκBα ( f ), activation of AKT and PTEN expression level ( g ). ( h ) A20 cells transduced with lentiviruses containing control or NEDD4shRNAs were stimulated with CD40L. At the indicated times, cell lysates were immunoprecipitated (IP) with CD40 antibody and the co-precipited proteins were analysed by immunoblotting with the indicated antibodies. ( i ) Control or NEDD4shRNAs A20 cells were transfected with vector, shRNA-resistant NEDD4 (Flag-resNEDD4) or NEDD4 E3 ubiquitin ligase-dead mutant (Flag-resNEDD4Mut) as indicated. After 36 h, cell lysates were collected after CD40L stimulation for the indicated times and the expression of Flag-resNEDD4 and Flag-resNEDD4/Mut and AKT activation were examined by immunoblotting. p-, phosphorylated. Data are representative of at least three independent experiments. Full size image As rapid ubiquitination of CD40 signalling components is critical for transducing effector signals [5] , the constitutive interaction of the E3 ligase NEDD4 with CD40 may ensure the temporal and spatial regulation of the ubiquitination process. Before we investigated the possible role of NEDD4 in CD40-associated ubiquitination reactions, we first made sure that NEDD4 is indeed involved in CD40 signalling. To do so, we examined CD40-mediated signals in Nedd4 − / − primary CD43 − B cells. Because Nedd4 − / − mice die perinatally, we generated fetal liver chimeras lacking Nedd4 only in haematopoietic cells, and isolated primary CD43 − B cells from the spleen of such mice ( Supplementary Fig. 3 ). As shown in Fig. 1e–g and Supplementary Fig. 4, although Nedd4 deletion had no effect on CD40L-induced activation of canonical and non-canonical NF-κB and MAPK pathways, the absence of NEDD4 almost abolished CD40L-induced AKT activation. Previously, reports suggested that NEDD4 might modulate phosphatase and tensin homolog (PTEN) ubiquitination and degradation [23] , [24] , other reports argued against the role of NEDD4 in PTEN stability [21] , [25] . In our study, we also failed to detect any noticeable difference between PTEN protein level in Nedd4 +/+ and PTEN protein level Nedd4 − / − B cells ( Fig. 1g ). It has also been reported that NEDD4 is involved in the regulation of some growth factor receptors signalling by controlling receptor stability [22] . However, in our study, we found that CD40 protein level was not affected by Nedd4 deletion ( Supplementary Fig. 3a ). In addition, knockdown of NEDD4 expression had no effect on the CD40L-induced recruitment of TRAF2 and TRAF3 in response to CD40L ( Fig. 1h ). These results indicated that NEDD4 is specifically and selectively involved in CD40-mediated AKT activation ( Fig. 1 and Supplementary Figs 4 and 5 ). More importantly, the defect of CD40-mediated AKT signalling caused by NEDD4 knockdown could be rescued by wild-type NEDD4 but not its ubiquitin E3 ligase-dead mutant, suggesting that the ubiquitin E3 ligase activity is essential for NEDD4 to function in CD40-mediated AKT signalling ( Fig. 1i ). NEDD4 promotes TRAF3 K63-linked ubiquitination To explore how NEDD4 regulates CD40-mediated AKT activation, we investigated whether NEDD4 is involved in any of the ubiquitination reactions associated with CD40 signalling. As both TRAF2 and TRAF3 ubiquitination are detected within minutes following CD40L treatment [5] , we tested whether TRAF2 or TRAF3 is potential substrate for NEDD4. To do so, we transfected haemagglutinin (HA)-TRAF2 or HA-TRAF3 with or without Myc-ubiquitin and Flag-NEDD4 plasmids into 293T cells. As shown in Fig. 2a , ubiquitination of TRAF3 but not TRAF2 was obviously increased in the presence of NEDD4. Importantly, when the amount of transfected NEDD4 was increased, the TRAF3 ubiquitination was elevated in a NEDD4 dose-dependent manner ( Fig. 2b ). Expression of ligase-dead NEDD4 mutant failed to show any effect on TRAF3 ubiquitination ( Fig. 2b ), strongly suggesting that TRAF3 is a potential substrate of NEDD4. This possibility was further supported by our finding that NEDD4 preferentially interacts with TRAF3 relative to TRAF2, and that the protein–protein interaction domain of NEDD4, WW repeats, is responsible for its interaction with TRAF3 ( Supplementary Fig. 6a,b ). 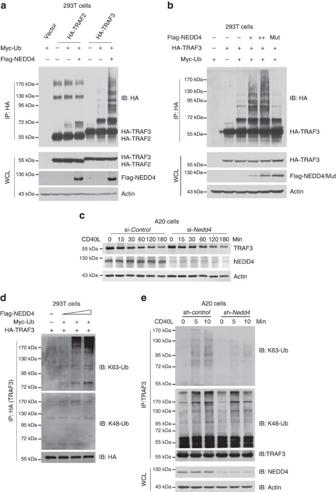Figure 2: NEDD4 promotes TRAF3 K63-linked ubiquitination upon CD40 engagement. (a) 293T cells were transfected with Myc-tagged Ubiquitin (Myc-Ub), HA-TRAF2, HA-TRAF3 and Flag-NEDD4 as indicated. Cell lysates were immunoprecipitated (IP) with anti-HA. Immune complexes were gel-separated and immunoblotted with anti-HA. (b) 293T cells were transfected with Myc-Ub, HA-TRAF3, increasing doses of Flag-NEDD4 or Flag-NEDD4 ligase-dead mutant (Mut) as indicated. Cell lysates were immunoprecipitated (IP) with anti-HA and the immune complexes were immunoblotted with anti-HA. (c) A20 cells transfected with control or NEDD4 short interfering RNAs were stimulated with CD40L. At the indicated times, cell lysates were prepared and immunoblotted with antibodies to TRAF3, NEDD4 and α-tubulin. (d) 293T cells were transfected with Myc-Ub, HA-TRAF3 and Flag-NEDD4 as indicated. After 36 h, cell lysates were prepared and immunoprecipitated with anti-HA, stringently washed and analysed by immunoblotting with linkage-specific antibodies recognizing K48- and K63-linked polyubiquitin. (e) A20 cells transduced with lentiviruses containing control or NEDD4 shRNAs were stimulated with CD40L. At the indicated times, cell lysates were prepared and immunoprecipitated with anti-TRAF3 and the immune complexes were stringently washed and immunoblotted with linkage-specific antibodies recognizing K48- and K63-linked polyubiquitin. Data are representative of at least three independent experiments. Figure 2: NEDD4 promotes TRAF3 K63-linked ubiquitination upon CD40 engagement. ( a ) 293T cells were transfected with Myc-tagged Ubiquitin (Myc-Ub), HA-TRAF2, HA-TRAF3 and Flag-NEDD4 as indicated. Cell lysates were immunoprecipitated (IP) with anti-HA. Immune complexes were gel-separated and immunoblotted with anti-HA. ( b ) 293T cells were transfected with Myc-Ub, HA-TRAF3, increasing doses of Flag-NEDD4 or Flag-NEDD4 ligase-dead mutant (Mut) as indicated. Cell lysates were immunoprecipitated (IP) with anti-HA and the immune complexes were immunoblotted with anti-HA. ( c ) A20 cells transfected with control or NEDD4 short interfering RNAs were stimulated with CD40L. At the indicated times, cell lysates were prepared and immunoblotted with antibodies to TRAF3, NEDD4 and α-tubulin. ( d ) 293T cells were transfected with Myc-Ub, HA-TRAF3 and Flag-NEDD4 as indicated. After 36 h, cell lysates were prepared and immunoprecipitated with anti-HA, stringently washed and analysed by immunoblotting with linkage-specific antibodies recognizing K48- and K63-linked polyubiquitin. ( e ) A20 cells transduced with lentiviruses containing control or NEDD4 shRNAs were stimulated with CD40L. At the indicated times, cell lysates were prepared and immunoprecipitated with anti-TRAF3 and the immune complexes were stringently washed and immunoblotted with linkage-specific antibodies recognizing K48- and K63-linked polyubiquitin. Data are representative of at least three independent experiments. Full size image As early reports showed that the K48-linked ubiquitination is critical for TRAF3 degradation upon CD40 engagement [5] , [12] , we next investigated whether NEDD4 contributes to this process. To our surprise, we found that NEDD4 knockdown did not influence the CD40L-induced TRAF3 degradation ( Fig. 2c ), indicating that NEDD4-mediated ubiquitination of TRAF3 does not contribute to its degradation. As several components of the CD40 signalling complex are subjected to both K48- and K63-linked ubiquitination upon CD40L treatment, we examined whether TRAF3 could also be ubiquitinated via a K63-linkage in response to CD40L stimulation. We detected CD40-mediated TRAF3 ubiquitination using K63- and K48-linked ubiquitination-specific antibody and found that TRAF3 is rapidly K63-linked ubiquitinated within 10 min after CD40 engagement, and the K63-linked ubiquitination could barely be detected 30 min after stimulation ( Supplementary Fig. 7 ). We then examined whether the NEDD4-mediated modification of TRAF3 is K63-linked ubiquitination. As shown in Fig. 2d , NEDD4-promoted TRAF3 ubiquitination was only recognized by a K63-linked ubiquitination-specific antibody, but not by a K48-linked ubiquitination-specific antibody. This result was further confirmed by mass spectrometry ( Supplementary Fig. 8 ). To test whether NEDD4 has the same effect on endogenous TRAF3 ubiquitination in CD40 signalling, we examined ubiquitination of TRAF3 following CD40L treatment in control and NEDD4shRNA A20 cells. Endogenous TRAF3 protein was immunoprecipitated and analysed by immunoblotting with K63- or K48-linked ubiquitination-specific antibodies. As shown in Fig. 2e , although TRAF3 was subjected to both K63- and K48-linked ubiquitination in response to CD40L treatment, only its K63-linked, but not K48-linked, ubiquitination was dramatically decreased in NEDD4shRNA A20 cells. These results suggested that NEDD4 promotes TRAF3 K63-linked ubiquitination upon CD40 engagement ( Fig. 2 and Supplementary Fig. 9 ). Most likely, the role of CD40 engagement in the reaction is to bring TRAF3 to the vicinity of NEDD4. TRAF3 K63-linked ubiquitination is required for CD40-AKT As deletion of NEDD4 only affects CD40-mediated AKT activation and NEDD4 mediates CD40L-induced K63-linked ubiquitination of TRAF3 ( Figs 1g and 2 ), we examined whether NEDD4-mediated K63-linked ubiquitination of TRAF3 is critical for CD40L-induced AKT activation. To do so, we first determined whether TRAF3 is essential for CD40L-induced AKT activation using Traf3 −/− mouse embryo fibroblasts (MEFs). Because CD40 is not expressed in MEFs, we established Traf3 +/+ and Traf3 −/− MEFs stably expressing CD40. As shown in Fig. 3a , CD40L potently induced AKT activation in CD40-expressing Traf3 +/+ cells but not in CD40-expressing Traf3 −/− cells, whereas CD40L-induced NF-κB alpha (IκBα) degradation was normal in the Traf3 −/− cells. The defect of AKT activation in Traf3 −/− cells is specific for CD40 signalling because epidermal growth factor-induced AKT activation was normal in these cells ( Fig. 3b ). In addition, CD40-mediated AKT activation is further elevated in Traf3 +/+ MEFs transduced with NEDD4-encoded lentivirus. But in Traf3 −/− MEFs, CD40-mediated AKT remains hardly activated even if NEDD4 was introduced ( Fig. 3c ). These results suggest NEDD4 is involved in CD40-AKT signalling through TRAF3. In addition, ligase-dead mutant of NEDD4 did not promote CD40L-induced AKT activation in MEF as wild-type NEDD4 did, suggesting that the elevation of CD40L-induced AKT activation caused by NEDD4 requires its E3 ligase activity ( Fig. 3d ). We analysed the NEDD4-catalysed ubiquitination sites of TRAF3 using liquid chromatography tandem mass spectrometry (LC-MS/MS). Two major sites, K369 and K513, were identified ( Fig. 3e ). We then generated a TRAF3 mutant in which both K369 and K513 were substituted with arginine residues and found that NEDD4-mediated K63-linked ubiquitination of TRAF3 mutant was decreased compared with wild-type TRAF3 ( Fig. 3f ). Importantly, when wild-type or mutant TRAF3 was introduced into CD40-expressing Traf3 −/− cells, only wild-type TRAF3, but not the mutant, restored CD40L-induced AKT activation ( Fig. 3g ). Thus, TRAF3 K63-linked ubiquitination mediated by NEDD4 is essential for CD40L-induced AKT activation. 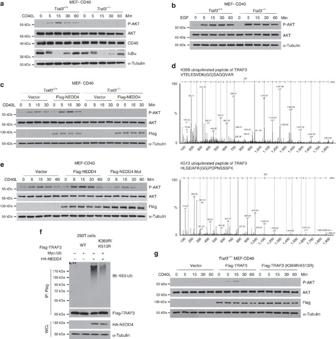Figure 3: NEDD4-mediated TRAF3 K63-linked ubiquitination is essential for CD40-mediated AKT signalling. (a,b) CD40-expressingTraf3+/+andTraf3−/−MEFs were stimulated with CD40L (a) or epidermal growth factor (236-EG-01M, R&D systems) (b). At the indicated times, cell lysates were collected and AKT activation was examined. (c) CD40Traf3+/+and CD40Traf3−/−MEFs were transfected with vector or Flag-NEDD4 and stimulated with CD40L for the indicated times. Cell lysates were collected and the expression of Flag-NEDD4 and AKT activation was examined. (d) CD40Traf3+/+MEFs were transfected with vector, Flag-NEDD4 or Flag-NEDD4 ligase-dead mutant (Mut) as indicated and stimulated with CD40L for the indicated times. Cell lysates were collected and the expression of Flag-NEDD4, Flag-NEDD4Mut and AKT activation was examined. (e) 293T cells were transfected with Myc-Ub, Flag-TRAF3 and HA-NEDD4. After 36 h, cell lysates were prepared and immunoprecipitated with anti-Flag. The immune complexes were subjected to LC-MS/MS analysis. TRAF3 peptides ubiquinated at K369 and K513 were detected and sequenced using Masslynx Pepseq software (Waters). (f) 293T cells were transfected with Myc-Ub, Flag-TRAF3 or Flag-TRAF3 (K369R/K513R), and HA-NEDD4 as indicated. Cell lysates were collected and immunoprecipitated with anti-Flag beads and the immune complexes were immunoblotted with K63-linked polyubiquitin-specific antibody. (g) CD40Traf3−/−MEFs were transfected with vector, Flag-TRAF3 or Flag-TRAF3 (K369R/K513R) and stimulated with CD40L. Cell lysates were collected at the indicated times and AKT activation was examined by immunoblotting. p-, phosphorylated. Western blot data are representative of at least three independent experiments. Mass spectrometry results are representative of two independent experiments. Figure 3: NEDD4-mediated TRAF3 K63-linked ubiquitination is essential for CD40-mediated AKT signalling. ( a , b ) CD40-expressing Traf3 +/+ and Traf3 −/− MEFs were stimulated with CD40L ( a ) or epidermal growth factor (236-EG-01M, R&D systems) ( b ). At the indicated times, cell lysates were collected and AKT activation was examined. ( c ) CD40 Traf3 +/+ and CD40 Traf3 −/− MEFs were transfected with vector or Flag-NEDD4 and stimulated with CD40L for the indicated times. Cell lysates were collected and the expression of Flag-NEDD4 and AKT activation was examined. ( d ) CD40 Traf3 +/+ MEFs were transfected with vector, Flag-NEDD4 or Flag-NEDD4 ligase-dead mutant (Mut) as indicated and stimulated with CD40L for the indicated times. Cell lysates were collected and the expression of Flag-NEDD4, Flag-NEDD4Mut and AKT activation was examined. ( e ) 293T cells were transfected with Myc-Ub, Flag-TRAF3 and HA-NEDD4. After 36 h, cell lysates were prepared and immunoprecipitated with anti-Flag. The immune complexes were subjected to LC-MS/MS analysis. TRAF3 peptides ubiquinated at K369 and K513 were detected and sequenced using Masslynx Pepseq software (Waters). ( f ) 293T cells were transfected with Myc-Ub, Flag-TRAF3 or Flag-TRAF3 (K369R/K513R), and HA-NEDD4 as indicated. Cell lysates were collected and immunoprecipitated with anti-Flag beads and the immune complexes were immunoblotted with K63-linked polyubiquitin-specific antibody. ( g ) CD40 Traf3 −/− MEFs were transfected with vector, Flag-TRAF3 or Flag-TRAF3 (K369R/K513R) and stimulated with CD40L. Cell lysates were collected at the indicated times and AKT activation was examined by immunoblotting. p-, phosphorylated. Western blot data are representative of at least three independent experiments. Mass spectrometry results are representative of two independent experiments. Full size image As is often the case, cytokine-induced AKT activation is through phosphatidyl inositol 3-kinase (PI3K) [26] . Indeed, we found that CD40-mediated AKT activation was almost completely blocked by PI3K inhibitor Wortmannin ( Fig. 4a ). We also found that NEDD4 was required for CD40L-induced recruitment of the PI3K regulatory subunit p85 to CD40 complex ( Fig. 4b ). Data from previous study indicated that p85 associates with TRAF3, so we investigated whether NEDD4 has any effect on the interaction between p85 and TRAF3 (ref. 27 ). We found that NEDD4 does not interact with p85, but promotes the interaction between TRAF3 and p85, and the binding of p85 to TRAF3 correlated with the extent of TRAF3 ubiquitination ( Fig. 4c,d ). 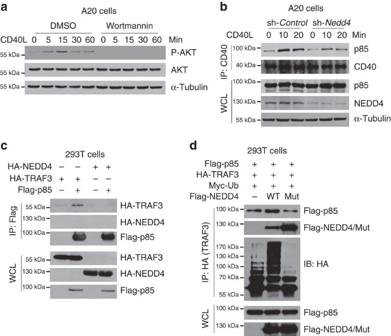Figure 4: NEDD4 promotes recruitment of p85 to TRAF3. (a) A20 cells pretreated with dimethylsulphoxide (DMSO) or 100 nM Wortmannin (681675, Calbiochem) for 1 h were stimulated with CD40L for the indicated times. Cell lysates were collected and AKT activation was examined by immunoblotting. (b) Control or NEDD4shRNAs A20 cells were stimulated with CD40L. At the indicated times, cell lysates were immunoprecipitated (IP) with CD40 antibody and the co-precipited p85 was analysed by immunoblotting. (c) 293T cells were transfected with HA-TRAF3 or HA-NEDD4 and Flag-p85 as indicated. After 36 h, immunopreciptation was performed using anti-Flag. Immune complexes and cell lysates were analysed by immunoblotting with anti-Flag and anti-HA. (d) 293T cells were transfected with Flag-p85, HA-TRAF3, Myc-Ub and Flag-NEDD4 or Flag-NEDD4 E3 ligase-dead mutant as indicated. After 36 h, immunopreciptation was performed using anti-HA. Immune complexes and cell lysates were analysed by immunoblotting with anti-Flag and anti-HA as indicated. p-, phosphorylated. Western blot data are representative of at least three independent experiments. Figure 4: NEDD4 promotes recruitment of p85 to TRAF3. ( a ) A20 cells pretreated with dimethylsulphoxide (DMSO) or 100 nM Wortmannin (681675, Calbiochem) for 1 h were stimulated with CD40L for the indicated times. Cell lysates were collected and AKT activation was examined by immunoblotting. ( b ) Control or NEDD4shRNAs A20 cells were stimulated with CD40L. At the indicated times, cell lysates were immunoprecipitated (IP) with CD40 antibody and the co-precipited p85 was analysed by immunoblotting. ( c ) 293T cells were transfected with HA-TRAF3 or HA-NEDD4 and Flag-p85 as indicated. After 36 h, immunopreciptation was performed using anti-Flag. Immune complexes and cell lysates were analysed by immunoblotting with anti-Flag and anti-HA. ( d ) 293T cells were transfected with Flag-p85, HA-TRAF3, Myc-Ub and Flag-NEDD4 or Flag-NEDD4 E3 ligase-dead mutant as indicated. After 36 h, immunopreciptation was performed using anti-HA. Immune complexes and cell lysates were analysed by immunoblotting with anti-Flag and anti-HA as indicated. p-, phosphorylated. Western blot data are representative of at least three independent experiments. Full size image NEDD4 regulates immunoglobulin class switch through AKT CD40 is a major in vivo inducer of immunoglobulin class switch, which is essential for humoral immunity. In primary B cells, AKT activation suppresses the initiation and frequency of immunoglobulin class switch, in part through the phosphorylation and inactivation of the Forkhead Box family (FOXO) member FOXO1 (refs 16 , 28 , 29 ). To further explore the biological significance of NEDD4 in CD40-mediated AKT signalling, we assessed FOXO1 phosphorylation mediated by CD40 activation in Nedd4 +/+ and Nedd4 − / − primary CD43 − B cells. As shown in Fig. 5a , CD40L-induced FOXO1 phosphorylation was obviously decreased in Nedd4 − / − cells compared with Nedd4 +/+ cells. CD40L-induced phosphorylation of FOXO3, another FOXO family AKT substrate, was also decreased. Overexpression of NEDD4 but not NEDD4 ligase-dead mutant upregulates CD40L-induced FOXO1 phosphorylation in MEF-CD40 cells ( Supplementary Fig. 10 ). It has been reported that phosphorylation of the FOXO1 by AKT induces its nuclear export and consequent inactivation of transcriptional activity. We then isolated cytoplasm and nuclear fractions of Nedd4 +/+ and Nedd4 −/− B cells, and examined the presence of FOXO1 in these fractions. Following CD40L treatment, the nuclear presence of FOXO1 was decrease in Nedd4 +/+ cells, but unchanged in Nedd4 −/− cells ( Fig. 5b ). Furthermore, in A20 cells, we found that the defect of CD40-mediated FOXO1 phosphorylation caused by NEDD4 knockdown could be rescued by wild-type NEDD4 but not its E3 ligase-dead mutant ( Fig. 5c ). These results suggest that the AKT-FOXO1 axis is defective in Nedd4 − / − B cells. 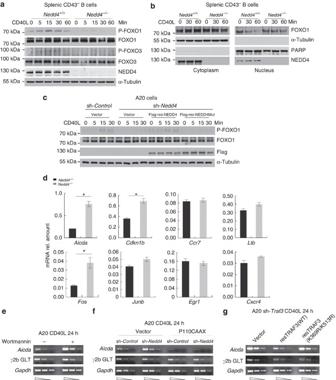Figure 5: NEDD4 regulates CD40-stimulated immunoglobulin class switch. (a) Primary CD43–splenic B cells were isolated from radiation chimeras reconstituted withNedd4+/+andNedd4−/−fetal liver stem cells and stimulated with CD40L. Cell lysates were collected at the indicated times, FOXO1 and FOXO3 phosphorylation were examined by immunoblotting. (b) Control or NEDD4shRNAs A20 cells were treated with CD40L for indicated times, cytoplasmic and nuclear protein were extracted and FOXO1 was analysed with immunoblotting. (c) Control or NEDD4shRNAs A20 cells were transfected with vector, shRNA-resistant NEDD4 (Flag-reNEDD4) or NEDD4 E3 ubiquitin ligase-dead mutant (Flag-reNEDD4Mut) as indicated. After 36 h, cell lysates were collected after CD40L stimulation for the indicated times. The expression of Flag-resNEDD4 and Flag-resNEDD4Mut and FOXO1 phosphorylation was examined by immunoblotting. (d)Nedd4+/+andNedd4−/−primary CD43–splenic B cells were stimulated with CD40L for 18 h. Total cellular RNA was extracted and mRNA amount of the indicated genes were analysed by qRT–PCR. The genes and their products wereAicda, AID;Cdkn1b, p27;Ccr7, CCR7;Ltb,lymphotoxin-β;Fos, c-Fos;Junb, JunB;Egr1, Egr-1;Cxcr4, CXCR4. *P<0.05 (two-tailed Student’st-test). Data are representative of three independent experiments and bars represent mean (±s.e.m.). (e–g) Semiquantitative PCR analysis ofAicda. (e) Wortmannin-treated or non-treated A20 cells were stimulated with CD40L for 24 h, total mRNAs were extracted andAicdaexpression was analysed. (f) sh-controlor sh-Nedd4A20 cells were transfected with vector or p110CAAX as indicated for 24 h, and stimulated with CD40L for 24 h. Total mRNAs were extracted andAicdaexpression was analysed. (g) sh-Traf3A20 cells were transfected with vector, Flag-TRAF3 and Flag-TRAF3 K369R/K513R mutant as indicated, then stimulated with CD40L for 24 h. Total mRNAs were extracted andAicdaexpression was analysed. Figure 5: NEDD4 regulates CD40-stimulated immunoglobulin class switch. ( a ) Primary CD43 – splenic B cells were isolated from radiation chimeras reconstituted with Nedd4 +/+ and Nedd4 −/− fetal liver stem cells and stimulated with CD40L. Cell lysates were collected at the indicated times, FOXO1 and FOXO3 phosphorylation were examined by immunoblotting. ( b ) Control or NEDD4shRNAs A20 cells were treated with CD40L for indicated times, cytoplasmic and nuclear protein were extracted and FOXO1 was analysed with immunoblotting. ( c ) Control or NEDD4shRNAs A20 cells were transfected with vector, shRNA-resistant NEDD4 (Flag-reNEDD4) or NEDD4 E3 ubiquitin ligase-dead mutant (Flag-reNEDD4Mut) as indicated. After 36 h, cell lysates were collected after CD40L stimulation for the indicated times. The expression of Flag-resNEDD4 and Flag-resNEDD4Mut and FOXO1 phosphorylation was examined by immunoblotting. ( d ) Nedd4 +/+ and Nedd4 −/− primary CD43 – splenic B cells were stimulated with CD40L for 18 h. Total cellular RNA was extracted and mRNA amount of the indicated genes were analysed by qRT–PCR. The genes and their products were Aicda , AID; Cdkn1b , p27; Ccr7 , CCR7; Ltb, lymphotoxin-β; Fos , c-Fos; Junb , JunB; Egr1 , Egr-1; Cxcr4 , CXCR4. * P <0.05 (two-tailed Student’s t -test). Data are representative of three independent experiments and bars represent mean (±s.e.m.). ( e – g ) Semiquantitative PCR analysis of Aicda . ( e ) Wortmannin-treated or non-treated A20 cells were stimulated with CD40L for 24 h, total mRNAs were extracted and Aicda expression was analysed. ( f ) sh- control or sh- Nedd4 A20 cells were transfected with vector or p110CAAX as indicated for 24 h, and stimulated with CD40L for 24 h. Total mRNAs were extracted and Aicda expression was analysed. ( g ) sh -Traf3 A20 cells were transfected with vector, Flag-TRAF3 and Flag-TRAF3 K369R/K513R mutant as indicated, then stimulated with CD40L for 24 h. Total mRNAs were extracted and Aicda expression was analysed. Full size image We further examined the expression of some downstream effectors of CD40 signalling with quantitative reverse transcription PCR (qRT–PCR; Fig. 5d ). We found that the mRNA expression of activation-induced cytidine deaminase (AID, Aicda ), the initiator of immunoglobulin class switch, was significantly upregulated in Nedd4 − / − B cells. qRT–PCR analysis also showed that the expression of p27 ( cdkn1b ) and c-Fos ( Fos ) was upregulated in Nedd4 − / − B cells. Other genes encoding transcription factor JunB ( Junb ), immediate early gene Egr-1 ( Egr1 ), cytokine lymphotoxin-β (Ltb) and chemokine receptors CXCR4 ( Cxcr4 ) and CCR7 ( Ccr7 ) were not affected by Nedd4 deficiency. To further investigate the mechanism of the regulation of Aicda by NEDD4, we examined Aicda expression induced by CD40L using semiquantitative PCR in A20 cells. In A20 cells, a post-switch IgG + B-cell lymphoma cell line, no CD40L-induced post-switch transcripts (PSTs) could be detected. But notable CD40L-induced Aicda and IgG2b germ-line transcript (γ2b GLT) could be readily detected, indicating that the upstream signalling events leading to class switch is intact in these cells ( Supplementary Fig. 11 ) [30] . As shown in the Fig. 5e , when AKT was inhibited by PI3K inhibitor Wortmannin, the expression of Aicda was apparently upregulated. Knockdown of NEDD4 with short hairpin RNA (shRNA) led to elevated Aicda expression. When a constitutive active PI3K (p110CAAX) was introduced, NEDD4 knockdown did not increase Aicda expression ( Fig. 5f , Supplementary Fig. 12a ). These results suggest that NEDD4 regulates Aicda expression through PI3K-AKT. Furthermore, when TRAF3 knockdown cells were reconstituted with wild-type TRAF3, the Aicda expression was inhibited, but the reconstitution of TRAF3 K369R/K513R mutant did not lead to the same inhibition ( Fig. 5g , Supplementary Fig. 12b,c ). These data suggest that NEDD4-mediated TRAF3 K63-linked ubiquitination has a role in the regulation of Aicda expression. To investigate whether the elevated Aicda induction in Nedd4 − / − B cells results in increased immunoglobulin class switch, we performed an in vitro class switch assay. As shown in Fig. 6a and Supplementary Fig. 13, class switch to IgG1 and IgG2a/2b triggered by CD40L was significantly increased in Nedd4 − / − B-cell compared with Nedd4 +/+ B cells, whereas class switch to IgG1 by lipopolysaccharide was not significantly affected. When AKT was inhibited by Wortmannin, Nedd4 knockout did not further increase CD40L-induced class switch ( Fig. 6b , Supplementary Fig. 14 ). We next investigated whether NEDD4 affects class switch in vivo . As shown in Fig. 6c , when Nedd4 +/+ and Nedd4 − / − B cells were transplanted into B-cell-deficient mice (μMT), higher level of total and keyhole limpet hemocyanin (KLH)-specific IgG was detected in the sera of Nedd4 − / − B cell-transplanted mice after 14 days of immunization with protein antigen KLH. These results suggest that NEDD4 is a B-cell-intrinsic regulator of immunoglobulin class switch. 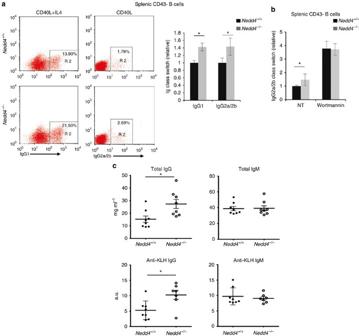Figure 6: NEDD4 affects class switchin vivo. (a) Flow cytometry of the immunoglobulin class switch inNedd4+/+andNedd4−/−B cells.Nedd4+/+andNedd4−/−primary CD43–splenic B cells incubated with CD40L (IgG2a/2b) or CD40L plus IL-4 (IgG1) for 4 days, and membrane IgG2a/2b- or IgG1-positive cells were measured with flow cytometry. Flow cytometry profiles are representative of four independent experiments. Bar graph shows the mean (±s.e.m.) folds of percent IgG+ cell inNedd4−/−B cells (grey bars) compared with that inNedd4+/+B cells (black bars). *P<0.05 (two-tailed Student’st-test). (b)Nedd4+/+andNedd4−/−primary CD43–B cells incubated with CD40L for 4 days in the absence and presence of Wortaminnin, and IgG2a/2b-positive cells were measured with flow cytometry. Bar graph shows the mean (±s.e.m.) folds of percent IgG+cell compared with that in non-treatedNedd4+/+B cells. (c) ELISA of total and KLH-specific IgG and IgM in sera of μMT mice reconstituted withNedd4+/+(filled circle) orNedd4−/−(open circle) B cells and immunized with KLH. Data were obtained 14 days after immunization. Each symbol represents one mouse; small horizontal bars indicate the mean values, error bar (±s.e.m.). *P<0.05 (two-tailed Student’st-test). AU, arbitrary unit; p-, phosphorylated. Data are representative of at least three independent experiments. Figure 6: NEDD4 affects class switch in vivo . ( a ) Flow cytometry of the immunoglobulin class switch in Nedd4 +/+ and Nedd4 −/− B cells. Nedd4 +/+ and Nedd4 −/− primary CD43 – splenic B cells incubated with CD40L (IgG2a/2b) or CD40L plus IL-4 (IgG1) for 4 days, and membrane IgG2a/2b- or IgG1-positive cells were measured with flow cytometry. Flow cytometry profiles are representative of four independent experiments. Bar graph shows the mean (±s.e.m.) folds of percent IgG+ cell in Nedd4 −/− B cells (grey bars) compared with that in Nedd4 +/+ B cells (black bars). * P <0.05 (two-tailed Student’s t -test). ( b ) Nedd4 +/+ and Nedd4 − / − primary CD43 – B cells incubated with CD40L for 4 days in the absence and presence of Wortaminnin, and IgG2a/2b-positive cells were measured with flow cytometry. Bar graph shows the mean (±s.e.m.) folds of percent IgG + cell compared with that in non-treated Nedd4 +/+ B cells. ( c ) ELISA of total and KLH-specific IgG and IgM in sera of μMT mice reconstituted with Nedd4 +/+ (filled circle) or Nedd4 −/− (open circle) B cells and immunized with KLH. Data were obtained 14 days after immunization. Each symbol represents one mouse; small horizontal bars indicate the mean values, error bar (±s.e.m.). * P <0.05 (two-tailed Student’s t -test). AU, arbitrary unit; p-, phosphorylated. Data are representative of at least three independent experiments. Full size image CD40 signalling is necessary for the development of B-cell immunity, including immunoglobulin class switch. Like other TNFR superfamily members, CD40 trimerizes after ligand binding and recruits multiple adaptors to form a receptor complex, which is essential for the downstream signal transduction. Although many aspects of CD40 signalling have been elucidated, the mechanism of CD40L-induced AKT activation remains elusive. Our study identified the HECT family E3 ubiquitin ligase NEDD4 as a previously unknown component of the CD40 signalling complex ( Supplementary Fig. 15 ). Unlike previously described components of the CD40 complex, which are recruited upon CD40 engagement, NEDD4 interacts with CD40 constitutively. NEDD4 promotes K63-linked ubiquitination of TRAF3 after TRAF3 is recruited to CD40 complex. Importantly, we found that NEDD4-mediated K63-linked ubiquitination of TRAF3 is critical for CD40L-induced AKT activation. Normally, components of the CD40 signalling complex are believed to be recruited to the receptor upon ligand engagement. In experiments originally designed to identify new components that are recruited to CD40 after its ligation, we identified NEDD4 repeatedly in immune complexes purified with a CD40 antibody using different immunoprecipitation strategies. However, the interaction between CD40 and NEDD4 was found to be ligand independent. A functional study using Nedd4 −/− B cells further confirmed that NEDD4 is a new component of the CD40 signalling complex required for AKT activation through ligand-induced TRAF3 K63-linked ubiquitination. Perhaps, the type of regulation ensures that TRAF3 is rapidly ubiquitinated upon its recruitment into the CD40 signalling complex. NEDD4 has been reported to be involved in various biological processes as an E3 ubiquitin ligase. Although early reports suggested that NEDD4 may catalyse both K48- and K63-linked ubiquitination, a recent structural study demonstrated that the E3 ubiquitin ligase activity of NEDD4 is more likely to be K63 specific [31] . Consistent with this result, we found that NEDD4 predominantly promotes K63-linked polyubiquitination of TRAF3. K48-linked ubiquitination and proteasomal degradation of TRAF3 was previously identified as an important mechanism of CD40L-induced non-canonical NF-κB activation. Whether TRAF3 could also be ubiquitinated via a K63-linkage in response to CD40L stimulation was not thoroughly investigated before. Here we report that TRAF3 is rapidly K63-linked ubiquitinated within 5 min after CD40 engagement. The K63-linked ubiquitination of TRAF3 is transient and could barely be detected 30 min after stimulation ( Fig. 2e , Supplementary Fig. 7 ). Although an early study implied that TRAF3 may be involved in CD40-mediated AKT activation, the detailed regulation of this process was not fully understood [27] . In our study, we found that NEDD4 ubiquitinated TRAF3 on K369 and K513, and this K63-linked ubiquitination of TRAF3 is essential for CD40L-induced AKT activation. Aicda encodes 198aa-protein AID that initiates class switch by deaminating deoxycytosines in single-stranded DNA and supercoiled double-stranded DNA. Aicda is hardly detectable in resting mature B cells, and could be induced by stimulations such as CD40L (T-cell dependent) and Toll-like receptors agonist (T-cell independent). Aicda expression level critically determines the level of class switch [32] . It was reported that FOXO1 exerts an essential function in class switch by upregulating Aicda expression. However, how does FOXO1 regulate Aicda expression and class switch is not clear [16] , [28] . One of the major functions of CD40 signalling is to mediate immunoglobulin class switch, which is essential for establishment of adaptive immunity [33] . Our findings suggest that NEDD4 functions as a fine-tuner of this process through TRAF3 K63-linked ubiquitination and AKT activation. Notably, NEDD4 is also involved in T-cell activation and T-helper cell function [20] . It will be of interest to determine whether NEDD4-catalysed TRAF3 K63-linked ubiquitination is also involved in the regulation of T-cell function. Generation of Nedd4 –/– fetal liver chimeras The Nedd4 gene trap insertional allele was generated by inserting a gene-trapping vector into intron 25 of Nedd4 , which results in disruption of this gene [21] . Fetal liver cell suspensions from Nedd4 +/+ and Nedd4 –/– embryos at days 14.5 were transferred by injection into tail veins of lethally irradiated (950 rad) 8-week-old male C57BL/6 recipients [20] . All mice were maintained in a specific pathogen-free barrier facility, and all experiments were performed on animals 8–20 weeks old. All animal experiments were approved by the Institutional Animal Care and Use Committee at the Beijing Institute of Basic Medical Sciences, China National Center of Biomedical Analysis. Splenic B-cell isolation and culture Mouse spleen was placed on 75 μM cell strainer (DKW33-N25, DAKEWE Biotech) and dissociated with the broad flat end of the plunger of syringe. Splenic total lymphocytes were obtained using mouse lymphocyte isolation kit (DKW33-R0100, DAKEWE Biotech). Primary CD43 – B cells were isolated by removing CD43 + cells with mouse CD43(Ly-48) magnetic beads (130-049-801, Miltenyi Biotec) and MS Columns (130-042-201, Miltenyi Biotec) according to the manufacturer’s protocol. B cells were cultured in RPMI medium 1640 supplemented with 10% fetal bovine serum (FBS), 50 μM β-mercaptoethanol, 100 U ml − 1 penicillin and 100 μg ml − 1 streptomycin at 37 °C under 5% CO 2 . B-cell survival and proliferation assay Purified B cells in replicate wells of 96-well plates (1 × 10 5 cells per well) were stimulated at 37 °C with Recombinant Mouse CD40L (0.5 μg ml −1 ; R&D systems; 1163-CL). In survival assay, BD Cell Viability Kit was used to count live cells, which were cultured for 4 days in medium alone or stimulated with CD40L. In proliferation assay, Nedd4 +/+ and Nedd4 –/– B cells were labeled with CFSE (Beyotime, C0051) and stimulated with CD40L for 4 days. B-cell transfer 2 × 10 6 primary Nedd4 +/+ or Nedd4 –/– CD43 – B cells were transferred into 8- to 10-week-old male B-cell-deficient mice (μMT, Jackson Laboratory) by injection into tail vein. Mouse immunization and serum immunoglobulin measurement Mice were injected subcutaneously with 100 μg KLH (H7017, Sigma) and 100 μl complete Freund’s Adjuvant (120022, Chondrex). Fourteen days after immunization, sera were collected and serum immunoglobulin level was measured by ELISA (eBioscience). Plasmids and stable cell lines Myc-Ub, HA-TRAF2 and HA-TRAF3 were cloned into pXJ40 vector. Flag-TRAF3 and Flag-TRAF3 (K369R/K513R) were cloned into pcDNA3 vector. Flag-NEDD4 and Flag-NEDD4-C867S were kindly provided by Reinhild Prange (Johannes Gutenberg-Universität Mainz, Germany). Flag-reNEDD4 and Flag-reNEDD4-C867S were sub-cloned from Flag-NEDD4 and Flag-NEDD4-C867S. Flag-p85 was cloned into pcDNA3 vector. GST-NEDD4, GST-NEDD4-C2, GST-NEDD4-WW1-WW4 and GST-NEDD4-HECT were constructed by inserting truncated NEDD4 into pGEX-KG vector. CD40 was cloned into MSCV-IRES-GFP retroviral vector. MEF were transfected with retrovirus and CD40-expressing cells were obtained by fluorescence-activated cell sorting. In vitro immunoglobulin class switch CD43 – B cells were cultured in the presence of 0.5 μg ml − 1 of CD40L (R&D) for IgG2a/2b, and for IgG1 class switch, 20 ng ml − 1 of recombinant murine IL-4 (214-14, Peprotech) was added. After 4 days in culture, IgG subclasses were measured by flow cytometry. Purified Rat Anti-Mouse CD16/CD32 (553141, BD Pharmingen) was used as blocker and Biotin Rat Anti-Mouse IgG1 (553441, BD Pharmingen / ), Biotin Rat Anti-Mouse IgG2a/2b (553398, BD Pharmingen) and FITC Streptavidin (554060, BD Pharmingen) were used to stain cells. RNA interference and transduction Mouse Nedd4 and control short interfering RNAs were purchased from Thermo Scientific (Mouse Nedd4 siGENOME ON-TARGET plus Smart Pool LU-058562-00-0010; Mouse control siGENOME ON-TARGET plus Smart Pool, Thermo Scientific Dharmacon). A 5′-TGCAGACCAGGCTGAGGAG-3′ oligonucleotide directed against mouse Nedd4 was cloned into pLSLPw lentiviral vector and lentivirus were prepared and packaged as described [6] . Cells were transduced with lentivirus in the presence of 5 μg ml − 1 polybrene (Sigma-Aldrich). After 36 h, the medium was replaced with selection medium containing 8 μg ml − 1 puromycin (EMD). Cells were cultured in 8 μg ml − 1 puromycin for 2 weeks before used for stimulation. Cell culture and transfection Mouse B-cell lymphoma A20 cells were obtained from American Type Culture Collection and cultured following the providers’ document [34] . A20 cells were transfected by electroporation with Amaxa Cell Line Nucleofector Kit V (DCV-1031, Lonza) and Nucleofector Device (Lonza). 293T cells and MEFs were cultured in DMEM containing 10% FBS and A20 cells were cultured in RPMI medium 1640 supplemented with 10% FBS, 50 μM β-mercaptoethanol at 37 °C in a humidified atmosphere of 5% CO 2 . 293T cells were transfected using VigoFect (Vigorous) and MEFs were transfected using Lipofectamine LTX Reagent (Invitrogen) following the manufacture’s instruction. Cell harvest and co-immunoprecipitation The total cell lysates were prepared in RIPA buffer containing 20 mM Tris-HCl pH 7.4, 150 mM NaCl, 10 mM EDTA, 1% (vol/vol) Triton X-100, 1% deoxycholate and protease inhibitor cocktail (04-693-132-001, Roche). For co-immunoprecipitation experiments, 293T cells were lysed in E1A buffer (50 mM HEPES pH 7.5, 250 mM NaCl, 0.1% Nonidet P-40, 5 mM EDTA) and protease inhibitor cocktail, and A20 cells were lysed in M2 buffer (20 mM Tris-HCl pH 7.5, 0.5% Nonidet P-40, 250 mM NaCl, 3 mM EDTA, 3 mM EGTA). The whole-cell homogenates were centrifuged and the supernatants were incubated with antibodies and rotated at 4 °C overnight, then incubated with protein A or protein G sepharose (GE Healthcare Life Sciences) for another 2 h. Immunoprecipitants were washed five times, and then boiled in loading buffer and subjected to SDS–polyacrylamide gel electrophoresis. qRT–PCR Cells were collected and the total RNA was extracted with Trizol (Invitrogen). The diluted RNA was reverse transcripted and analysed with SYBR Premix Ex TaqTM II (Perfect Real Time; DRR081A, TAKARA) and 7300 Real-Time PCR System (Applied Biosystems). The primers listed in Supplementary Table 2 were used to amplify the specific fragment of gene transcripts. Gapdh was used for normalization. Semiquantitive RT–PCR Total RNA was purified with Trizol A20 cells according to the manufacturer’s instructions (Invitrogen). The diluted RNA was reverse transcripted to cDNA. Serially diluted cDNA was used for 30 cycles of PCR with primer pairs of Aicda, Gapdh, GLTs and PSTs. For PCR of GLTs, the following primers were used: (μ) ImF and CmR; (γ3) Ig3F and Cg3R; (γ1) Ig1 and Cg1R; (γ2b) Ig2bF Cg2bR; (γ2a) Ig2aF and Cg2aR; (ε) IeF and CeR; and (α) IaF and CaR. For PCR of PSTs, the following primers were used: (γ3) ImF and Cg3R; (γ1) ImF and Cg1R; (γ2b) ImF and Cg2bR; (γ2a) ImF and Cg2aR; (ε) ImF and CeR; and (α) ImF and CaR. The primers listed in Supplementary Table 3 were used to amplify the specific fragment of gene transcripts. Ubiquitination analysis Cell lysates were prepared in RIPA lysis buffer. Cell lysates were sheared with sonication and centrifuged at 12,000 r.p.m. for 10 min. SDS was added into the supernatants to a final concentration 1%, noncovalently associated proteins were removed by boiling at 95 °C for 7 min. Then the samples were diluted to 0.1% SDS and were immunoprecipitated overnight at 4 °C with antibody and protein A/G sepharose beads (GE Healthcare Life Sciences). The immunoprecipitants were washed five times with lysis buffer and boiled in loading buffer and subjected to SDS–polyacrylamide gel electrophoresis, followed by immunoblotting with rabbit Anti-Ubiquitin-Lys48 (clone Apu2, 05-1307, Merck Millipore), Anti-Ubiquitin-Lys63 (clone Apu3, 05-1308, Merck Millipore) and a light chain-specific HRP-Mouse-anti-Rabbit IgG (211-032-171, Jackson ImmunoResearch) or light-chain specific HRP-Goat-anti-Mouse IgG (115-035-174, Jackson ImmunoResearch). For MS analysis, Flag-TRAF3 was eluted with 3 × FLAG PEPTIDE (F4799, Sigma-Aldrich) in elution buffer (50 mM Na-HEPES pH7.4, 150 mM NaCl) for 30 min. The eluted sample was ultrafiltrated, washed and concentrated with 0.5 ml Amicon Ultra-centrifugal filters (UFC501024, Millipore). Mass spectrometry In-solution and in-gel digestion were carried out according to a previously published protocol [35] . The digested samples were analysed by nanoLC-MS/MS (nanoACQUITY UPLC and SYNAPT G2 HD mass spectrometer, Waters). Mass spectrometry data were acquired with Data Dependent Analysis mode, processed with PLGS 2.4 software (Waters), and the resulting peak list was searched against the NCBI database with the MASCOT search engine, de novo sequencing were performed using Masslynx Pepseq 4.1 software (Waters). Antibodies and Reagents Antibodies specific to phosph-p38 (Thr180/Tyr182) (9211, Cell Signaling Technology); CD40 (sc-975, Santa Cruz Biotechnology; Supplementary Fig. 2a ); NEDD4 (2740, Cell Signaling Technology); TRAF3 (sc-947 and sc-6933, Santa Cruz Biotechnology); FOXO1 (1874-1, EPITOMICS), Phospho-FOXO1(Ser256) (9461, Cell Signaling Technology); FOXO3a (2497, Cell Signaling Technology); phosph-FOXO3a (ser253) (13129, Cell Signaling Technology); HA-probe Antibody (sc-7392 and sc-805, Santa Cruz Biotechnology); purified Rat Anti-Mouse CD43 (Ly-48, Leukosialin) Monoclonal Antibody (553268, BD Pharmingen); rabbit IgG (sc-2027, Santa Cruz Biotechnology), p85 (06-496, Merck Millipore, dilution 1:5,000); α-tubulin (T5168, Adam Equipment, dilution 1:10,000); JNK (9252, Cell Signaling Technology); phosph-JNK (Thr183/Tyr185) (9251, Cell Signaling Technology); NF-κB p65 (C-20) (sc-372, Santa Cruz, dilution 1:5,000); Phospho-IκBα (Ser32) (2859, Cell Signaling Technology); IκBα (C-21) (SC-371, Santa Cruz); TRAF2 (Clone 324522) (MAB3277, R&D Systems); P100/P52 (4882, Cell Signaling Technology); Phospho-AKT(Ser473) (9271, Cell Signaling Technology); AKT (9272, Cell Signaling Technology); Recombinant epidermal growth factor (236-EG-01M, R&D systems); Wortmannin (681675, Calbiochem); lipopolysaccharide (L2880, Sigma); Syndecan-1 (142509, BioLegend); B220 (103207, BioLegend). Antibody dilution for western blotting is 1:1,000 unless indicated otherwise. Full western blots can be found in Supplementary Fig. 16 . Antibody dilutions for cell cytometry is 1:100 unless indicated otherwise. How to cite this article: Fang, D.-F. et al. NEDD4 ubiquitinates TRAF3 to promote CD40-mediated AKT activation. Nat. Commun. 5:4513 doi: 10.1038/ncomms5513 (2014).